Human monoclonal antibodies targeting the haemagglutinin glycoprotein can neutralize H7N9 influenza virus The recently identified avian-originated influenza H7N9 virus causes severe pulmonary disease and may lead to death in humans. Currently, treatment options for the prevention and control of fatal H7N9 infections in humans remain limited. Here we characterize two human monoclonal antibodies (HuMAbs), HNIgGA6 and HNIgGB5, by screening a Fab antibody phage library derived from patients who recovered from H7N9 infection. Both antibodies exhibit high neutralizing activity against H7N9 virus in cells. Two amino acids in the receptor-binding site, 186V and 226L, are crucial for the binding of these two HuMAbs to viral haemagglutinin antigens. Prophylaxis with HNIgGA6 and HNIgGB5 confers significant immunity against H7N9 virus in a mouse model and significantly reduces the pulmonary virus titre. When administered post infection, therapeutic doses of the HuMAbs also provide robust protection against lethality. These antibodies might represent a potential alternative or adjunct to H7N9 pandemic interventions. In February 2013, an outbreak caused by the avian-originated influenza A virus H7N9 subtype was reported in eastern China [1] . Patients presented with fever, cough, sputum production and shortness of breath, and severe cases were characterized by rapidly progressive pneumonia, respiratory failure, acute respiratory distress syndrome and even death [2] . Within a few months, the virus had resulted in 137 infection cases, including 45 fatalities [3] . The outbreak caused a severe threat to public health, and H7N9 became a great concern. Influenza A viruses are enveloped RNA viruses of the family Orthomyxoviridae. These viruses possess eight negative-sense genomic segments and are classified into subtypes based on two surface glycoproteins, haemagglutinin (HA) and neuraminidase (NA). To date, 16 HA (H1-H16) and 9 NA (N1-N9) subtypes have been identified in avian natural reservoirs. A newly identified influenza A virus from little yellow-shouldered bats was designated as H17N10 (refs 4 , 5 ). A similar virus genome, H18N11, was identified in the flat-faced fruit bat [6] . Several subtypes have adapted to humans and have caused pandemics, such as the H5N1 (ref. 7 ) outbreak, the H9N2 infection [8] and the H7N7 outbreak in the Netherlands in 2003 (ref. 9 ) and the global H1N1 outbreak [10] . However, the outbreak in China represents the first time that a H7N9 virus was recognized as infectious and fatal to humans. H7N9 viruses are resistant to the M2-ion channel blockers known as amantadine and rimantadine, which have been widely utilized as anti-influenza drugs. Laboratory testing confirmed that H7N9 is sensitive to NA inhibitors, such as oseltamivir and zanamivir [11] , [12] . However, treatment options for human patients remain limited. Moreover, H7N9 may acquire genetic changes, rendering one or more influenza antiviral drugs less effective [11] , [12] , as with seasonal influenza viruses. New preventative and therapeutic strategies are urgently needed to combat human H7N9 infections. Neutralization by an antibody is one of the most important mechanisms by which hosts defend themselves against viral infections, and the protection provided by neutralizing antibodies against varicella, hepatitis A, hepatitis B, rabies and respiratory syncytial virus has been clinically effective [13] . There has also been benefit from using transfused blood, serum and blood products in the treatment of influenza A virus. Transfusion of human blood products from patients recovering from the 1918 pandemic in Spain reduced mortality by 50% (ref. 14 ). Recently, by screening human combinatorial antibody libraries and immortalized memory B cells, many human antibodies against different influenza A viruses have been isolated [15] , [16] , [17] , [18] . Some of these antibodies exhibit neutralizing activity and can prophylactically or therapeutically suppress the virus in experimentally infected animals. In this study, we generated a Fab antibody phage library derived from patients who recovered from H7N9 infections. To obtain a comprehensive understanding of the antibody repertoire in H7N9 patients, we screened the library with purified H7N9 virions. A large number of monoclonal antibodies (MAbs) targeting different viral antigens were obtained, and two MAbs possessing high neutralizing activity against live H7N9 virus were investigated. Epitope identification demonstrated that the receptor-binding site (RBS) was critical for MAbs binding to the virus. Two single amino-acid residue substitutions in the RBS, V186G and L226Q (H3 numbering), led to the loss of antibody binding. We applied the antibodies for prophylactic and therapeutic immunization in a mouse model to protect against H7N9 challenge. Both antibodies exhibited potent antiviral effects and prevented viral infection. To the best of our knowledge, this is the first report describing human monoclonal antibodies (HuMAbs) against the newly found H7N9 virus. The HuMAbs identified in this study may shed light on the development of effective H7N9 pandemic vaccines and have potential for use in the treatment of H7N9 infection. Generation of H7N9-specific antibodies We established two Fab phage display libraries (for λ and κ light chains) from the peripheral blood mononuclear cells of convalescent patients infected with H7N9. These two phage libraries contained 1.2 × 10 8 and 1.7 × 10 8 independent clones, respectively. After three rounds of panning, 1,536 colonies were picked randomly, and 816 positive Fab clones were identified. Sequence analysis of the 816 positive Fab clones revealed 18 unique clones. Among these 18 Fabs, 6 derived from the V H 3 family, and 12 derived from the V H 4 family. The light chains of these Fabs are derived from the lambda gene family V λ 1 and the kappa gene families V κ 1, V κ 2 and V κ 3. 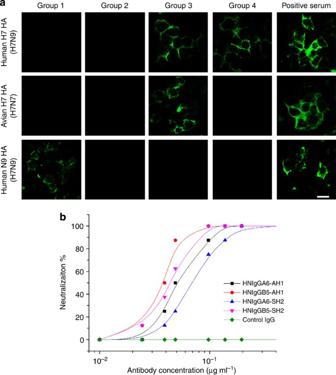Figure 1: General features and neutralizing activity of the MAbs. (a) The binding activity of the MAbs to HA and NA proteins were determined using IFA. Representative results are shown. The IFA results are representative of three independent replicates; scale bar, 10 μm. (b) The neutralizing activities of HNIgGA6 and HNIgGB5 were tested on cells. An anti-HIV human IgG was used as a negative control. According to their sequences, the antibodies can be divided into four groups ( Table 1 ). Group 1 includes V H 3 and V λ 1, group 2 includes V H 4 and V λ 1, group 3 includes V H 3 and V κ 3, and group 4 includes V H 4 and V κ 1. Table 1 Classification of the selected anti-H7N9 Fab gene fragments from human anti-H7N9 Fab antibody library Full size table General features and neutralizing activity of the MAbs The immunospecificity of all MAbs was tested by ELISA in 96-well microtitre plates coated with inactivated H7N9 virions and the viral proteins HA and NA. An avian H7 HA protein and bovine serum albumin (BSA) were used as controls. 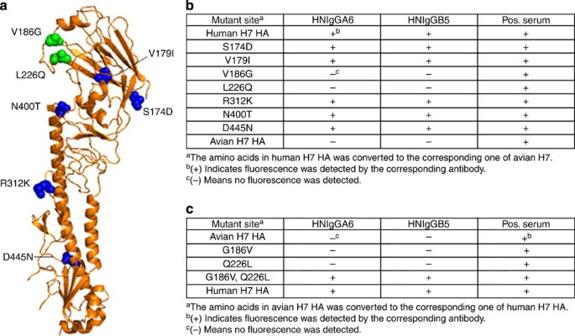Figure 2: Epitope mapping for HNIgGA6 and HNIgGB5. (a) All seven amino-acid substitutions in HA protein between human H7 HA and avian H7 are labelled on the HA structure (PDB accession code4BSA). The residues in the RBS region are in green, and the others are in blue. (b,c) The mutated HA protein was expressed in cells and detected using IFA. The IFA results are representative of three independent replicates. Pos., positive. Although all of the MAbs reacted with H7N9 virions, the MAbs from group 1 exhibited NA-binding activity; group 3 MAbs were able to interact with both human and avian H7 HA; and group 4 MAbs recognized human H7 HA but not avian H7 ( Table 2 ). To further characterize the binding specificities of the 18 MAbs, we expressed viral HA and NA proteins in 293T cells. The binding affinity of these proteins with the MAbs was tested using immunofluorescence assay (IFA). The results were consistent with those obtained using ELISA detection: group 1 MAbs recognized H7N9 NA protein; group 2 MAbs did not directly interact with HA or NA; group 3 MAbs bound to both human and avian H7 HA and group 4 MAbs reacted with only human H7 HA. Representative results are shown in Fig. 1a . Table 2 Binding activities of all 18 unique Fabs with H7N9 antigen Full size table Figure 1: General features and neutralizing activity of the MAbs. ( a ) The binding activity of the MAbs to HA and NA proteins were determined using IFA. Representative results are shown. The IFA results are representative of three independent replicates; scale bar, 10 μm. ( b ) The neutralizing activities of HNIgGA6 and HNIgGB5 were tested on cells. An anti-HIV human IgG was used as a negative control. Full size image Because all 18 Fabs reacted with either H7N9 virions or antigens, their neutralizing effect against the virus was tested. Group 4 MAbs exhibited noticeable neutralizing activity against H7N9 virus on cells; however, neutralizing activity was rarely detected for group 3 antibodies; and no detectable neutralizing activity was found for group 1 or group 2 antibodies ( Table 1 ). In group 4, two Fabs exhibited stronger neutralizing activity and were converted into full-length IgG1 molecules named HNIgGA6 (derived from H7N9Fab12) and HNIgGB5 (derived from H7N9Fab17) for further study. To test the reactivity of the two HuMAbs, a HA inhibition (HI) assay was performed. Both HuMAbs exhibited potent HI activity. The HI titre for HNIgGA6 was as low as 0.8 μg ml −1 , compared with 1.6 μg ml −1 for HNIgGB5. Their neutralizing activity against live H7N9 virus was then determined on cells. H7N9 virus was incubated with serially diluted HuMAbs and then used to infect MDCK cells. Virus-induced cytopathic effect (CPE) was observed until 3 days post infection (d.p.i.). The neutralizing activity of the HuMAbs against H7N9 (A/Shanghai/2/2013, -SH2) was also tested. As shown in Fig. 1b , both HNIgGA6 and HNIgGB5 were able to neutralize H7N9 virus in a dose-dependent manner. Epitope mapping Because both Fabs bound to human H7 HA but not to avian H7 in the IFA and ELISA assays, it is plausible that the MAbs distinguish between the two HA proteins. As shown in Fig. 2a , there are seven amino-acid substitutions between human H7 HA and avian H7 HA. We then constructed seven mutants of human H7 HA, each time changing one of the seven amino acids to the corresponding amino acid in avian H7 HA. All mutants were detected. Nevertheless, only V186G or L226Q abolished the binding activity with both HuMAbs ( Fig. 2b ). To further confirm these findings, the avian H7 HA was reversely mutated at the same position. The constructs were also expressed in cells and detected by IFA. As expected, the reversal in binding activity was only restored when both mutations G186V and Q226L were introduced into avian H7 HA ( Fig. 2c ). Escape mutants were also selected by culturing H7N9 virus in MDCK cells in the presence of serial tenfold dilutions of HuMAb as described previously [19] . After five passages, stable variants were obtained for both HuMAbs, which grew at similar levels in the presence and absence of the antibody, and no inhibitory effect was seen in HI tests. The entire HA gene was sequenced. As expected, amino-acid substitutions were detected. Interestingly, the substitutions occurred at the same positions, V186G and L226Q, which are identical to the residues of avian H7 HA. These results together indicated that the epitope for HNIgGA6 and HNIgGB5 is dependent on the residues at positions 186 and 226. Figure 2: Epitope mapping for HNIgGA6 and HNIgGB5. ( a ) All seven amino-acid substitutions in HA protein between human H7 HA and avian H7 are labelled on the HA structure (PDB accession code 4BSA ). The residues in the RBS region are in green, and the others are in blue. ( b , c ) The mutated HA protein was expressed in cells and detected using IFA. The IFA results are representative of three independent replicates. Pos., positive. Full size image Prophylactic efficacy of HNIgGA6 and HNIgGB5 in mice To explore the prophylactic efficacy of the HuMAbs, BALB/c mice were passively immunized with either HNIgGA6 or HNIgGB5 at 1, 5 and 10 mg kg −1 . The mice were then challenged with 50 μl of 10 × LD 50 of H7N9 virus 24 h later. A control group, which immunized with an irrelevant control human IgG, was also infected. Death and body weight changes in the mice were monitored. As shown in Fig. 3a , animals that received an irrelevant control antibody succumbed to infection in 4–11 days after viral challenge. In contrast, almost all preparations of HNIgGB5 or HNIgGA6 conferred 100% protection from lethality by H7N9 in the infected mice, with the exception of 1 mg kg −1 HNIgGA6, which was only partially (60%) protective for the mice ( Fig. 3a ). Animals immunized with an irrelevant control antibody rapidly lost weight ( Fig. 3b ). However, although mice receiving HNIgGB5 and HNIgGA6 also lost weight after infection, body weight was gradually restored at approximately 5 d.p.i. and even increased by the study’s end ( Fig. 3b,c ), with the exception of the group treated with 1 mg kg −1 HNIgGA6, which lost approximately 30% of body weight. These results demonstrated that both HNIgGB5 and HNIgGA6 substantially decreased the mortality and morbidity of mice infected with H7N9. To investigate serum half-life, the pharmacokinetic behaviour of the HuMAbs was evaluated in mice. Six mice per group were administered 200 μg HNIgGA6 or HNIgGB5 via intraperitoneal injection. Blood samples were then collected, and the concentrations of HNIgGA6 and HNIgGB5 in mice were determined. As shown in Fig. 3d , the average half-life of the HNIgGA6 was 6.5±0.9 days and that of HNIgGB5 was 6.8±0.5 days. 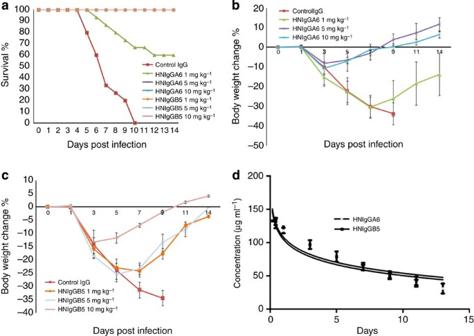Figure 3: Prophylactic efficacy of HNIgGA6 and HNIgGB5 in mice. Mice received HNIgGA6 or HNIgGB5 24 h before H7N9 infection and were monitored daily for 14 days. (a) The survival rate is presented (n=15 per group). (b,c) The average body weight change of the mice is shown (n=15 per group). (d)In-vivohalf-life of the HuMAbs was determined (n=6 per group). Results inb–dare presented as the mean±s.d. Figure 3: Prophylactic efficacy of HNIgGA6 and HNIgGB5 in mice. Mice received HNIgGA6 or HNIgGB5 24 h before H7N9 infection and were monitored daily for 14 days. ( a ) The survival rate is presented ( n =15 per group). ( b , c ) The average body weight change of the mice is shown ( n =15 per group). ( d ) In-vivo half-life of the HuMAbs was determined ( n =6 per group). Results in b – d are presented as the mean±s.d. Full size image Histopathology detection Previous reports of experimentally induced infection in mouse models have indicated that the H7N9 virus is able to disseminate to lung tissues after infection, where it replicates actively [20] . To verify that the protection of the infected mice was due to the inhibition of viral proliferation, viral dissemination in the lungs was determined. As shown in Fig. 4a , mice that received an irrelevant human IgG constantly had high titres of virus in the lungs from 1 to 7 d.p.i. ( Fig. 4a ). In contrast, with passive immunization by either HNIgGA6 or HNIgGB5, viral proliferation was substantially inhibited, and virus titres were difficult to be detected at 7 d.p.i. ( Fig. 4a ). Because H7N9 influenza virus usually induces severe alveolitis in infected mice, pathological changes in the lung tissue were further examined. As shown in Fig. 4b , mice that received prophylaxis with HNIgGA6 and HNIgGB5 not only had lower viral titres in the lung but also had lower pathology scores compared with the control group. Less dramatic pathological changes in the lungs are also shown in Fig. 4c–e . In the control group, H7N9 infection induced severe peribronchiolitis, perivasculitis, interstitial pneumonitis and alveolitis in the mice ( Fig. 4c ). In the HNIgGA6-treated group, the mice showed less interstitial pneumonitis and alleviated peribronchiolitis ( Fig. 4d ). Signs of perivasculitis and peribronchiolitis also decreased in the mice that were immunized with HNIgGB5 ( Fig. 4e ). 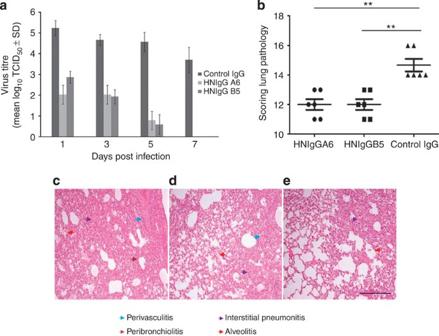Figure 4: Histopathological detection. Mice were passively immunized with HNIgGA6, HNIgGB5 or the control human IgG for 24 h and then challenged with a lethal dose of H7N9 virus. (a) Pulmonary virus titres were determined at indicated times. Virus titres were substantially reduced in the HuMAb-treated groups (P<0.05,t-test). (b) Histopathological changes in the lungs were scored. Less dramatic pathological changes in the lungs of the HuMAb-treated mice compared with the control group were detected (P<0.05,t-test). Results ina,bare presented as the mean±s.d. (n=6 per group). (c–e) Histopathology of pulmonary tissue from H7N9-infected mice. Scale bar, 200 μm. Control human IgG-treated mice (c). Mice immunized with HNIgGA6 (d) or HNIgGB5 (e). Figure 4: Histopathological detection. Mice were passively immunized with HNIgGA6, HNIgGB5 or the control human IgG for 24 h and then challenged with a lethal dose of H7N9 virus. ( a ) Pulmonary virus titres were determined at indicated times. Virus titres were substantially reduced in the HuMAb-treated groups ( P <0.05, t -test). ( b ) Histopathological changes in the lungs were scored. Less dramatic pathological changes in the lungs of the HuMAb-treated mice compared with the control group were detected ( P <0.05, t -test). Results in a , b are presented as the mean±s.d. ( n =6 per group). ( c – e ) Histopathology of pulmonary tissue from H7N9-infected mice. Scale bar, 200 μm. Control human IgG-treated mice ( c ). Mice immunized with HNIgGA6 ( d ) or HNIgGB5 ( e ). Full size image Therapeutic treatment against H7N9 infection in mice To better understand the clinically relevant effect of antiviral therapy against H7N9 infection, BALB/c mice were infected with 50 μl of 10 × LD 50 of H7N9 for 3 h and then passively immunized with either HNIgGA6 or HNIgGB5. The efficacy of the treatment was determined. As shown in Fig. 5a , all mice in the control group died within 10 days after virus infection, whereas HNIgGB5 was able to protect mice against a lethal challenge of H7N9 virus; this protection varied with dose. When using 5 mg kg −1 of HNIgGB5, 53% of the infected mice survived, and therapeutic treatment with 20 mg kg −1 of HNIgGB5 prevented mortality in 93% of mice ( Fig. 5a ). When using 5–20 mg kg −1 of HNIgGA6, 47–60% of the infected mice survived ( Fig. 5a ). The body weight of the infected mice was recorded. Similar to previous results, mice in the control group gradually lost body weight after virus challenge and succumbed to virus infection ( Fig. 5b ); however, after immunization with either HNIgGA6 or HNIgGB5, all of the infected mice started to regain their body weight at approximately 5–7 d.p.i., suggesting an improvement in health. The therapeutic efficacy of HNIgGB5 was further tested in BALB/c mice that had been infected with 50 μl of 10 × LD 50 of H7N9 for 24 h. Similar to previous results, 20 mg kg −1 of HNIgGB5 was able to prevent mortality in 80% of mice ( Fig. 5c ). Passive immunization with HNIgGB5 at 24 h post infection (h.p.i.) was also able to improve the health of infected mice, as suggested by the gradual recovery of body weight ( Fig. 5d ). To determine the possibility of the emergence of escape mutants in the mice after passive immunization, 30 dead mice (15 from the HNIgGA6-treated group and 15 from the HNIgGB5-treated group) were collected. Viruses were recovered from lung tissue by propagation in MDCK cells for 72 h and were then subjected to a virus neutralization assay. Viruses were obtained from 19 dead mice, and all remained neutralizable by both antibodies. No noticeable difference in the neutralization titre was found compared with the native H7N9 virus. The lung tissues of the 30 dead mice were then mixed together for viral RNA extraction. The entire HA gene was amplified and cloned for sequencing. A total of 400 colonies were sequenced. Random amino-acid substitutions were detected, and most were distant from the RBS. However, two mutants bearing I182T and L226Q close to the 190-α-helix were also identified, and these mutations might lead to the loss of neutralizing activity for the antibodies. 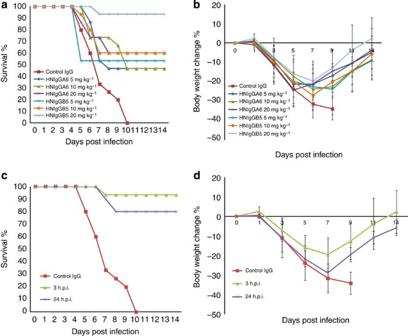Figure 5: Therapeutic treatment against H7N9 infection with HNIgGA6 and HNIgGB5 in mice. Mice were challenged with a lethal dose of H7N9 virus (n=15 per group). (a) The infected mice were immunized 3 h.p.i. with HNIgGA6 or HNIgGB5. The survival rate of the mice was monitored daily until 14 d.p.i. (b) Body weight changes were recorded daily for 14 days. (c) The infected mice were immunized 24 h.p.i. with 20 mg kg−1HNIgGB5. The survival rate of the mice was monitored daily until 14 d.p.i. (d) Body weight changes were also recorded daily for 14 days. Results inb,dare presented as the mean±s.d. Figure 5: Therapeutic treatment against H7N9 infection with HNIgGA6 and HNIgGB5 in mice. Mice were challenged with a lethal dose of H7N9 virus ( n =15 per group). ( a ) The infected mice were immunized 3 h.p.i. with HNIgGA6 or HNIgGB5. The survival rate of the mice was monitored daily until 14 d.p.i. ( b ) Body weight changes were recorded daily for 14 days. ( c ) The infected mice were immunized 24 h.p.i. with 20 mg kg −1 HNIgGB5. The survival rate of the mice was monitored daily until 14 d.p.i. ( d ) Body weight changes were also recorded daily for 14 days. Results in b , d are presented as the mean±s.d. Full size image The emergence of the H7N9 influenza A virus subtype caused a significant global health concern due to the severity of the infection and because it resulted in approximately 25% mortality in humans. A total of 454 H7N9 cases resulting in at least 171 deaths were reported by September 2014, and most cases were antigenically similar to the -AH1 isolate [21] . An effective antiviral therapy against H7N9 infection is urgently needed. Neutralizing antibodies can prevent viral infections, and recent studies with these antibodies have shown promise for the treatment of influenza A virus infections, including H1N1, H3N2 and H5N1 (refs 22 , 23 , 24 ), especially in sporadic human infections [25] . However, due to the high frequency of antigenic drift, most neutralizing antibodies recognize a limited clade or subtype of influenza virus. To the best of our knowledge, the only neutralizing antibody that has been reported to react with H7 is CR8020, which shows neutralizing activity against most group 2 influenza viruses [26] . Unfortunately, CR8020 has been less effective against the recent H7N9 virus [27] . In this study, we generated a combinatorial library with blood from patients recovering from H7N9 infection and screened this library for neutralizing antibodies. Two antibodies neutralized the H7N9 virus, both -AH1 and -SH2, in vitro and in vivo . To date, these strains are the only two candidate influenza vaccine viruses according to the World Health Organization [21] . These antibodies exhibit potential for the treatment of human pandemic or sporadic cases of zoonotic H7N9 influenza. During the H7N9 outbreak, over 75% of the documented human cases were caused by exposure to poultry; however, limited human-to-human transmission cannot be excluded in a few small clusters of human infection [1] , [28] . The adaptation of viruses to human transmission might involve multiple genetic factors; however, the receptor-binding properties of the HA glycoprotein are crucial. HA is a trimer of identical subunits, each of which contains two polypeptides that result from the proteolytic cleavage of a single precursor [29] . Each HA monomer contains a RBS in its globular head that is responsible for virus-receptor recognition and interaction, several conserved amino acids (98Y, 153W, 183H and 195Y), and three conserved secondary structure elements at its edges: the 130- and 220-loops and the 190-α-helix [29] , [30] . The receptor-binding specificity and affinity of the HA for H7N9 virus have been estimated using several methods. As a general rule, avian viruses prefer to bind sialic acid in an α2,3-linkage to galactose, whereas human viruses prefer to bind α2,6-linked sialic acid [31] , [32] . In addition to its role in receptor binding, HA also mediates entry of the genome-transcriptase complex into cells during infection by inducing membrane fusion through its stalk region [29] . No obvious sequence differences exist between human and avian H7 viruses that could influence virus pathogenicity [29] , [33] . Using IFA detection, we found that both of the identified HuMAbs interact with viral HA protein but not with NA. Further analysis revealed that the RBS motif is crucial for the binding of the neutralizing antibodies to HA. Either one of two amino-acid residue substitutions in the RBS, V186G or L226Q, resulted in a loss of human H7 HA-binding ability. In contrast, the reverse mutants, G186V and Q226L, endowed avian H7 HA with the ability to bind to the antibodies. These results, when taken together with those of the in-vivo and in-vitro escape mutant assay, demonstrated that the epitope for HNIgGA6 and HNIgGB5 is dependent on the RBS motif and residues at positions 186 and 226. Considering the essential roles of these two residues in virus-receptor binding [34] , [35] , it is plausible that the neutralizing antibodies, HNIgGA6 and HNIgGB5, bind to the HA protein through the RBS and interfere with its recognition of and interaction with the human cellular receptor. A previous report declared that neutralizing antibodies that recognize the globular head exhibit strong HI activity, whereas neutralizing antibodies that recognize the stalk region usually do not exhibit such activity [36] . Our results are consistent with these findings in that both HNIgGA6 and HNIgGB5 exhibit potent HI activity. In summary, characterization of the neutralizing antibodies provided further support for the essential roles of 186V and 226L in virus–receptor interactions. Moreover, these results provide insight for the development of novel neutralizing antibodies. The neutralizing antibody concentration required for viral neutralization is usually much lower for antibodies that react with the globular head than for antibodies that bind to the stalk region of the influenza virus [24] , [26] . Nevertheless, even though the HuMAbs described here that target the RBS of HA display high neutralizing activity and the essential roles played by 186V and 226L limit their variation and consequent antigenic drift, changes can occur in the RBS over time because of the widespread presence of H7N9 influenza in avian and poultry species and continuing zoonotic introductions into humans. In this regard, more HuMAbs, especially antibodies targeting distinct and more conserved epitopes, are needed for alternative and adjunctive treatments for H7N9 infection. BALB/c mice are highly susceptible to H7N9 infection [20] , [37] . H7N9 can be disseminated into multiple organs, including the brain, liver, spleen, kidney and intestine. Peak virus shedding from the respiratory tract is detected approximately 2 d.p.i. Viral infection typically leads to clinical signs including body weight loss, ruffled fur and death. We evaluated the anti-viral effects of the HuMAbs, HNIgGA6 and HNIgGB5, in a mouse model. Prophylaxis with HNIgGB5 at 1–10 mg kg −1 conferred 100% protection of the mice against H7N9 infection, and HNIgGA6 conferred to a lower level of protection. The health of the infected mice was also substantially improved, as indicated by body weight recovery. Further assessment demonstrated that passive immunity was associated with a falling viral load in the respiratory tract (lungs) for both HNIgGA6 and HNIgGB5, indicating that the limitation of H7N9-induced illness was due to the inhibition of viral proliferation. Histopathological detection also supported these findings. Prophylaxis with HNIgGA6 and HNIgGB5 noticeably prevented pathological changes of the lungs because of viral infection. In summary, prophylactic administration of HNIgGA6 or HNIgGB5 appeared beneficial by abolishing H7N9-mediated weight loss and pathological changes of lung tissue and allowed more rapid recovery of the infected animals. The therapeutic efficacy of the HuMAbs was then tested. Passive immunization of mice with HNIgGA6 or HNIgGB5 at 3 h.p.i. was also effective against H7N9 infection. Mice that received HNIgGA6 treatment (5–20 mg kg −1 ) exhibited a survival rate of 47–60%, and 93% of the mice that were treated with 20 mg kg −1 of antibody HNIgGB5 survived. The average body weight of the infected mice declined during the first 5d.p.i. However, as a benefit, the mice gradually recovered their body weight after treatment with the antibodies. HNIgGB5 exhibited a higher neutralizing activity in mice, although HNIgGA6 exhibited stronger in-vitro HI activity. When treated with 1 mg kg −1 HNIgGA6, 60% of the infected mice survived; in contrast, HNIgGB5 was able to protect 100% of the mice in the prophylaxis test. In addition, the highest survival rate obtained with HNIgGB5 was 93% when mice were immunized post infection with 20 mg kg −1 antibodies; this value compares with a 60% survival rate when treated with HNIgGA6. This might be explained by HNIgGB5 exhibiting better in-vivo accessibility than HNIgGA6 or to possible side effects caused by HNIgGA6 in mice due to the human origin of the antibodies. Most human H7N9 infections, especially zoonotic cases, are not treated by health care or drug therapy until at least several days after illness onset; thus, we tested the therapeutic efficacy of HNIgGB5 when used to immunize at 24 h.p.i. At a concentration of 20 mg kg −1 , the antibody was able to save 80% of the mice from a lethal dose of H7N9 virus infection. Taken together, these results demonstrate that both antibodies offer a very effective treatment against novel H7N9 infection in mice. However, additional tests using ferrets and other animal models are required to determine the potential efficacy and utility of passive immunity in humans. In addition, the effectiveness of the antibodies when inoculated even later after infection should be determined. In addition, because temporal cellular immune suppression and infection-mediated endogenous signals can interfere with the efficacy of exogenous HuMAbs, studies are needed to determine the optimum timing for antibody inoculation. H7N9 is resistant to the M2-ion channel blockers amantadine and rimantadine, which have been widely utilized as anti-influenza drugs. Recent studies have revealed that the virus can be inhibited by the NA inhibitors oseltamivir and zanamivir. Oseltamivir treatment, administered as long as 48 h or more after disease onset, was associated with a remarkable falling viral load in the respiratory tract in most patients with H7N9 infection [11] . This finding is encouraging and exciting. Unfortunately, a R292K mutation in NA (N9 numbering) that confers resistance to both oseltamivir and zanamivir was detected in 2 out of 11 patients tested, and one such mutation occurred within 7 days after oseltamivir therapy [11] . A R152K mutation was also detected during the test [11] . This mutation exhibits mild resistance to both zanamivir and oseltamivir in vitro [38] . Neutralizing antibodies such as HNIgGA6 and HNIgGB5 that attack the HA protein directly at residues 186V and 226L provide an alternative H7N9 treatment. Even if escape were possible, passive immunization would likely be highly effective when used in conjunction with other established therapies to reduce the prospect of viral escape or resistance. In summary, we identified and characterized two HuMAbs that possess potent neutralizing activity against H7N9 in vitro and in vivo . The HuMAbs recognize the RBS of the HA antigen at 186V and 226L and provided modest defenses against challenge with lethal doses of the H7N9 influenza in mice. The antibodies were generated in response to natural infectious H7N9 virus and have protected an individual. Furthermore, the antibodies are of human origin; thus, the risk of HuMAbs reacting with self-antigens is less than that present when antibodies are generated from other animals. The generation of such HuMAbs provides not only important insight into the protective immune response to H7N9 virus in humans but also represents a potential alternative treatment of H7N9 infection. Ethics and human subjects This study was reviewed and approved by the Ethics Committee of the Institute of Pathogen Biology at the Chinese Academy of Medical Sciences and Peking Union Medical College. Peripheral blood samples from H7N9 patients were collected by the Shanghai and Beijing Centers for Disease Control and Prevention. Written informed consent was obtained for the use of peripheral blood samples. Murine studies were performed in an animal biosafety level 3 facility using HEPA-filtered isolators. The experiment was performed in accordance with the Chinese national guidelines for the care of laboratory animals and was approved by the Institutional Animal Care and Use Committee of the Institute of Laboratory Animal Science at Peking Union Medical College (ILAS-PC-2013-008). All efforts were made to minimize animal suffering and to use the minimum number of animals. Three hundred and fifty female 6-week-old specific pathogen-free BALB/c mice (Institute of Laboratory Animal Sciences, Beijing, China) were used in this study. The animals weighed 16.0 g±2.0 g, and six to ten mice were housed in one individually ventilated cages (IVC) cage under controlled conditions of humidity (60±10%) and temperature (25±2 °C). Food and water were available ad libitum , and veterinarians skilled in the care and maintenance of mice supervised the animal care. Mice were euthanized using CO 2 asphyxiation followed by cervical dislocation. Cells and viruses Madin–Darby canine kidney (MDCK; American Type Culture Collection) and HEK293 T (293T; American Type Culture Collection) cells were maintained in Dulbecco's modified Eagle’s medium (DMEM; HyClone) supplemented with 10% fetal bovine serum (FBS; Invitrogen), 100 U ml −1 penicillin and 100 μg ml −1 streptomycin at 37 °C with 5% CO 2 . The H7N9 viruses used in this study were A/Anhui/1/2013 and A/Shanghai/2/2013 (provided by Shanghai Centers for Disease Control and Prevention). The H7N9 virus titres were determined as the median end-point of the tissue culture infectious dosage (TCID 50 ). Serially diluted virus samples (from 10 −2 to10 −9 ) were added to MDCK cells in 96-well plates, and the plates were then incubated for 3 days at 37 °C. The TCID 50 values were measured by determining CPE and were calculated using the Reed-Muench method [39] . Phage library construction Peripheral blood mononuclear cells were isolated from the peripheral blood of recovered patients 3–4 weeks after hospitalization. RNA was then extracted and purified from the lymphocytes using the RNeasy kit (Qiagen) according to the manufacturer’s protocol. cDNA was transcribed using total RNA as a template, Thermoscript reverse transcriptase (Invitrogen) as the enzyme and oligodT as a primer. The heavy and light chain genes were amplified from the cDNA using PCR and sequentially cloned into the phagemid vector pComb3H (kindly provided by the Scripps Research Institute). The anti-H7N9 phage antibody library was constructed using previously described primers and methods [40] . Selection of H7N9-specific Fabs The antibody library was screened by panning with purified H7N9 virions. After three rounds of panning, crude Fab antibody preparations were tested by indirect ELISA using 96-well plates coated with 50 ng per well of purified H7N9 virions. Horseradish peroxidase (HRP)-conjugated goat anti-human Fab (Sigma) was prepared at a 1:2,000 dilution to be used as the secondary antibody. The human Fab MAbs were purified on an anti-Fab affinity chromatography column for further characterization and functional analysis. The purity of the human Fab MAbs was confirmed using SDS–polyacrylamide gel electrophoresis analysis. ELISA with recombinant viral proteins and purified virions We utilized ELISA assays with H7N9 viral proteins and purified virions to identify the antigen for the MAbs. The recombinant proteins used in the ELISA assay were recombinant HA proteins from H7N9 and avian influenza H7N7 (A/chicken/Netherlands/1/03; Sino Biological) and recombinant NA protein from H7N9 (Sino Biological). The 96-well plates were coated overnight at 4 °C with 50 ng of purified H7N9 virions or 100 ng recombinant protein per well. After blocking with 2% BSA, the plates were incubated with individual MAbs at 100 ng per well at 37 °C for 1 h and then washed three times with phosphate-buffered saline containing 0.1% Tween-20. HRP-conjugated goat anti-human IgG antibody (Sigma) was prepared at a 1:2,000 dilution to be used as a secondary antibody; the plates were incubated at 37 °C for a further 1 h, and the reaction was developed using 3,3′,5,5′-tetramethylbenzidine (TMB) as the substrate. The absorbance at 450 nm was measured using an ELISA plate reader (Tecan). Expression of viral rHA and rNA proteins in cells For transient expression in 293T cells, HA and NA genes were cloned from H7N9 (A/Anhui/1/2013) and inserted into the vector pcDNA3.0 (Invitrogen) under cytomegalovirus promoter control. A Flag tag (DYKDDDDK) was tandemly anchored to the N- terminus of these proteins for western blotting detection. The nucleotide sequences of the plasmids and the orientation of the inserted fragments were verified by DNA sequencing. The HA of avian H7N7 (A/pigeon/Wenzhou/559/2013) was custom synthesized (GENEWIZ) and cloned into pcDNA3.0 as a control. Cells were transformed using Lipofectamine 2000 reagent (Invitrogen) following the manufacturer’s protocol. Immunofluorescence assay To measure the reactivity of the MAbs for viral antigens, rHA and rNA were transiently expressed in 293T cells. Cells were grown in 24-well plates and either directly stained in the wells or prepared as monolayers on glass slides and subjected to acetone fixation. The cells were then incubated with MAbs at 37 °C for 30 min. Bound antibodies were detected using FITC-conjugated goat anti-human IgG antibodies (Sigma) was prepared at a 1:100 dilution and then observed under a fluorescence microscope. IgG1 expression and purification Human IgG1 MAbs were expressed and purified as described previously [41] . Briefly, fully human IgG1 antibodies were constructed by cloning the heavy and light chain variable regions of H7N9-specific antibodies into PIGG vectors (provided by the Scripps Research Institute) for IgG1 heavy and light chain expression. IgG1 samples were produced from the PIGG vector by transiently transfecting human 293T cells using Lipofectamine 2000 (Invitrogen). The collected medium was purified by affinity chromatography using a recombinant Protein A HiTrap column (GE Healthcare). The purity of IgG1 was confirmed using SDS–polyacrylamide gel electrophoresis and ELISA. Haemagglutination inhibition H7N9 virus was diluted to 8 haemagglutinating units and incubated with an equal volume of serially diluted antibody at room temperature. An equal volume of 0.5% horse red blood cells (freshly collected by Institute of Laboratory Animal Sciences) was added to the wells, and incubation was continued on a gently rocking plate for 30 min at room temperature. Cell button formation was scored as evidence of HI. Neutralization assay MAbs were serially diluted in twofold steps in DMEM containing 2% FBS; the samples were then inactivated at 56 °C for 30 min. Next, 50 μl of 100 × TCID 50 viral sample was combined with each MAb and incubated at 37 °C for 1 h. The virus and MAb mixtures (total 100 μl) were added to MDCK cells in 96-well plates and further incubated for 2 h at 37 °C under 5% CO 2 . The plates were washed and replaced with DMEM containing tosylphenylalanylchloromethylketone-modified trypsin after incubation and scored for CPE after 3 days. The highest MAb dilution in which 50% of the MDCK cells were intact was scored as the neutralization titre. All experiments were performed under BSL-3 conditions. An anti-HIV human IgG (Immune Technology) was used as a negative control. Site-directed mutagenesis Mutagenic primers were designed for site-directed mutagenesis after aligning the sequences of the HA regions of H7N9 and avian H7N7. The primers are shown in Table 3 . The mutated DNA fragments of the HA gene of H7N9 were amplified using PCR, cloned into pCDNA3.0, and confirmed by DNA sequencing to exclude any secondary mutations. All constructs were transfected into 293T cells for transient expression. The resulting mutated rHAs were assayed using IFA as described above to assess the binding activity of the MAbs. Table 3 Mutagenic primers used in the study Full size table HuMAbs for prophylaxis and therapy in mice Female 6-week-old specific pathogen-free BALB/c mice were obtained from the Institute of Laboratory Animal Sciences, Beijing, China. To measure prophylactic efficacy, 15 mice per group (divided into three independent groups) were intraperitoneally injected with 1, 5 or 10 mg kg −1 of purified HuMAbs 24 h before being challenged intranasally with 50 μl of a 10 × LD 50 mouse infectious dose of H7N9 virus under anaesthesia with isoflurane. Another 15 mice that were immunized with a recombinant fusion protein corresponding to human IgG1 (Sino Biological) were also infected as controls. The mice were observed daily for signs of disease and mortality for up to 14 days. For therapy against H7N9, the mice (also 15 mice per group) were infected with 10 × LD 50 of H7N9; then, 3 or 24 h later, the mice were injected with 5, 10 or 20 mg kg −1 of purified HuMAbs and were observed daily for signs of disease and mortality for up to 14 days. Control human IgG-treated mice were infected in the same way and monitored every day. To avoid over-disturbing the mice, we weighed the mice every 2 days and only live mice were recorded. Pharmacokinetic detection To determine the in- vivo half-life of the HuMAbs, mice were given 200 μg of the antibodies via intraperitoneal injection. Blood (approximately 50 μl) was drawn from the tail plexus at each time point and processed to serum. The study duration was 13 days. The HuMAb concentrations were determined using ELISA. The plates were coated overnight at 4 °C with 50 ng of purified H7N9 virions per well. After blocking with 2% BSA, the plates were incubated with individual mouse serum dilutions at 37 °C for 1 h and then washed three times with phosphate-buffered saline containing 0.1% Tween-20. HRP-conjugated goat anti-human IgG antibody (Sigma, USA) was prepared at a 1:2,000 dilution to be used as a secondary antibody; the plates were incubated at 37 °C for a further 1 h, and the reaction was developed using TMB as substrate. The absorbance at 450 nm was measured using an ELISA plate reader (Tecan). Histopathology Six mice per group that received prophylaxis with either HNIgGA6 or HNIgGB5 (5 mg kg −1 ) were necropsied according to a standard protocol at 5 d.p.i. Naive human IgG-treated mice were also collected as controls. The lungs were fixed in 10% neutral buffered formaldehyde and embedded in paraffin. Tissue sections (5 μm) were stained with haematoxylin and eosin and analysed microscopically. Scoring of lung pathology was graded by a pathologist blinded to the experimental design on a scale described in previously published studies as follows [42] , [43] , [44] : peribronchiolitis (inflammatory cells, primarily lymphocytes surrounding a bronchiole), perivasculitis (inflammatory cells, primarily lymphocytes surrounding a blood vessel), interstitial pneumonitis (increased thickness of alveolar walls associated with inflammatory cells, primarily neutrophils) and alveolitis (inflammatory cells, primarily neutrophils and macrophages within alveolar spaces). Each histopathological change was scored on a scale of 0 (no change) to 4 (maximum inflammation), with a score of 4 being based upon our prior observations of maximal pathological changes induced by influenza virus infection of mouse lungs [45] . Statistical analysis The virus titre and scoring of lung pathology were evaluated independently for each of the infected mice. All results are presented as the mean±s.d. Statistical analysis was performed using SSPS (Statistical Package for the Social Sciences) 10.0 software. Differences with P <0.05 were considered statistically significant. How to cite this article: Chen, Z. et al . Human monoclonal antibodies targeting the haemagglutinin glycoprotein can neutralize H7N9 influenza virus. Nat. Commun. 6:6714 doi: 10.1038/ncomms7714 (2015).